Ecological succession of a Jurassic shallow-water ichthyosaur fall After the discovery of whale fall communities in modern oceans, it has been hypothesized that during the Mesozoic the carcasses of marine reptiles created similar habitats supporting long-lived and specialized animal communities. Here, we report a fully documented ichthyosaur fall community, from a Late Jurassic shelf setting, and reconstruct the ecological succession of its micro- and macrofauna. The early ‘mobile-scavenger’ and ‘enrichment-opportunist’ stages were not succeeded by a ‘sulphophilic stage’ characterized by chemosynthetic molluscs, but instead the bones were colonized by microbial mats that attracted echinoids and other mat-grazing invertebrates. Abundant cemented suspension feeders indicate a well-developed ‘reef stage’ with prolonged exposure and colonization of the bones prior to final burial, unlike in modern whale falls where organisms such as the ubiquitous bone-eating worm Osedax rapidly destroy the skeleton. Shallow-water ichthyosaur falls thus fulfilled similar ecological roles to shallow whale falls, and did not support specialized chemosynthetic communities. Whale carcasses create long-lived, ecologically significant habitats that support diverse and highly specialized ‘whale fall’ communities, and which may have been critical in the dispersal and evolution of chemosymbiotic communities during the Cenozoic [1] , [2] . Following their discovery, it was hypothesized that during the Mesozoic the carcasses of marine reptiles may have fulfilled similar roles and hosted analogous communities [3] , [4] , [5] . Despite its importance in understanding the early evolution of modern marine ecosystems, this hypothesis has yet to be rigorously tested. Few examples of marine reptile fall communities have been documented or studied in detail [3] , [6] and the only known chemosymbiotic community comprises micro-grazing provannid gastropods and ataphrid-like vetigastropods associated with two upper Cretaceous plesiosaurs from outer shelf and slope settings [7] . Community succession in modern whale falls has been first described in the deep sea (>200 m depth), where it has been divided into discrete ecological stages [8] , [9] . Following an initial ‘mobile scavenger stage’, when sharks and other organisms remove the flesh and soft tissues, an ‘enrichment opportunist’ stage develops with polychaetes, crustaceans and other small-sized opportunists thriving on the remaining whale organic matter. Next, a ‘sulphophilic stage’ in which the oxidation of inorganic compounds, such as sulphide or methane, derived from microbial degradation of the bone lipids supports a chemosynthetic community, including chemosymbiotic bivalves and free-living bacteria (for example, Beggiatoa ). Finally, a ‘reef stage’ has been hypothesized, in which the remaining skeleton is colonized by suspension feeders exploiting hard substrata and flow enhancement [8] . Recent time-series analyses have shown, however, that whale fall community succession is not always as linear as this simple model suggests: stages are not always discrete but may overlap each other, and many factors can influence their development, such as sedimentation, temperature and water depth [10] . Whale fall communities in shallow water are somewhat different from their deep-water counterparts because they experience more complex biostratinomic processes and support communities with lower endemicity [11] , [12] . It was thought that shallow whale falls did not develop a significant ‘sulphophilic stage’, but recent experiments have shown that it is possible for the chemosynthetic community to develop on outer shelf whale falls within 5 years [11] . Available data suggest that at whale falls, as in other localized habitats fuelled by reducing compounds such as hydrothermal vents and hydrocarbon seeps, there is a progressive increase in the importance of organic carbon derived from chemosynthesis moving from coastal to open marine settings, with heterotrophic communities dominating in shallow waters and autotrophic communities dominating at deep-sea sites [13] . In this paper, we report the first detailed study of ecological succession of a shallow-water ichthyosaur fall community from the Late Jurassic to test whether the carcass supported a similar community to that of fossil and recent whale falls. The Ichthyosauria were a diverse, cosmopolitan group of Mesozoic marine reptiles that ranged from the late Early Triassic (Olenekian) to the Late Cretaceous (Turonian) [14] , and some species reached lengths of 21 m [15] . Like many cetaceans, they were active predators fully adapted to aquatic life, capable of rapid sustained swimming and able to dive to depths of 500 m or more [16] . Ichthyosaur bones have a cancellous microstructure very similar to that of whales and dolphins [17] and likely also contained lipids within the marrow spaces [18] . In this study, we undertake a detailed palaeoecological analysis of an ichthyosaur fall community associated with a Late Jurassic Ophthalmosaurus skeleton, focusing on the fossil macroinvertebrates and fossil evidence of microbially mediated processes to reconstruct the successional stages that preceded final burial of the carcass. We show that this shallow-water ichthyosaur fall supported a very similar community succession to that of modern and fossil shallow-water whale falls. Geological context and recovery The studied specimen comprises the associated, disarticulated fossil remains of a single, ca. 3 m long, individual of the genus Ophthalmosaurus , found partly enclosed in large concretionary blocks ( Fig. 1 ). It comes from the upper part of the Ringstead Clay Member (Sandsfoot Formation, Upper Oxfordian), which consists of pale-to-dark grey, variably calcareous mudstones and was deposited in a shallow, low-energy, offshore shelf setting, characterized by low sedimentation rates [19] . All skeletal elements were disarticulated before final burial ( Fig. 1a ), possibly by both scavenging and current (storm?) activity, although most paddle elements were associated in broad clusters on either side of the concretionary blocks and a few vertebrae were found in loose association with their neural arches. Soon after excavation the specimen was partially prepared to preserve as much taphonomic information as possible [20] . 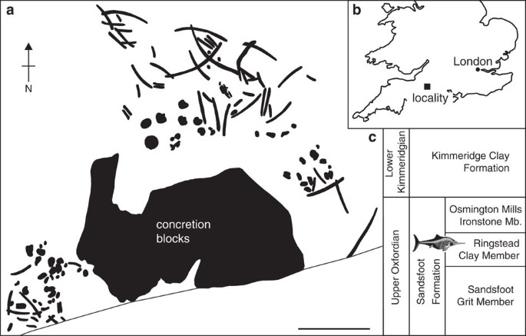Figure 1: Plan of the excavation, locality of recovery of theOphthalmosaurusand stratigraphy. (a) Plan view of theOphthalmosaurusremains at the recovery site. Bones are highly disarticulated. (b) Map showing the locality of recovery, Dorset, UK. (c) Stratigraphy. The specimen comes from the upper part of the Ringstead Clay Member of the Sandsfoot Formation, Upper Oxfordian in age. Figure modified with permission from the publisher ref.20. Scale bars, (a) 50 cm. Figure 1: Plan of the excavation, locality of recovery of the Ophthalmosaurus and stratigraphy. ( a ) Plan view of the Ophthalmosaurus remains at the recovery site. Bones are highly disarticulated. ( b ) Map showing the locality of recovery, Dorset, UK. ( c ) Stratigraphy. The specimen comes from the upper part of the Ringstead Clay Member of the Sandsfoot Formation, Upper Oxfordian in age. Figure modified with permission from the publisher ref. 20 . Scale bars, ( a ) 50 cm. Full size image Evidence of mobile scavengers and grazers Trace fossils preserved in concave epirelief on the surfaces of some of the bones are evidence of both scavenging and grazing ( Fig. 2 ). Scavenging is inferred by the presence of short (<1 cm), sharp, narrow grooves, with a U- or V-shaped cross-section, that are found individually or in subparallel clusters on the ribs ( Fig. 2a ). They resemble marks left by smooth-edged teeth of fish ( cf. , ref. 21 : Fig. 3e ), and their small size excludes the possibility that they were left by active predation on the live animal. 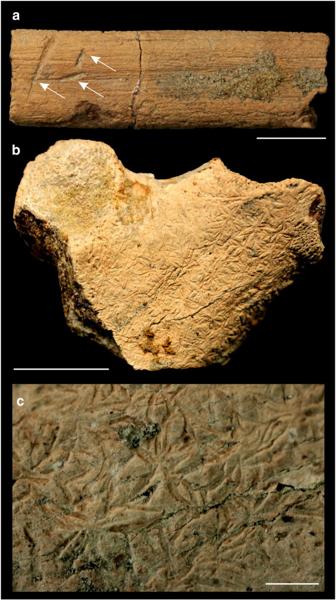Figure 2: Trace fossils on theOphthalmosaurusbones. (a) Rib showing sharp, narrow grooves (white arrows) probably left by the scavenging action of small fishes. (b)G. pentaxichnospecies on a fragmented proximal rib. (c) Detail of figurea; note the star shape of the trace fossil. Scale bars, (a) 0.5 cm; (b) 1 cm; (c) 0.2 cm. Figure 2: Trace fossils on the Ophthalmosaurus bones. ( a ) Rib showing sharp, narrow grooves (white arrows) probably left by the scavenging action of small fishes. ( b ) G. pentax ichnospecies on a fragmented proximal rib. ( c ) Detail of figure a ; note the star shape of the trace fossil. Scale bars, ( a ) 0.5 cm; ( b ) 1 cm; ( c ) 0.2 cm. 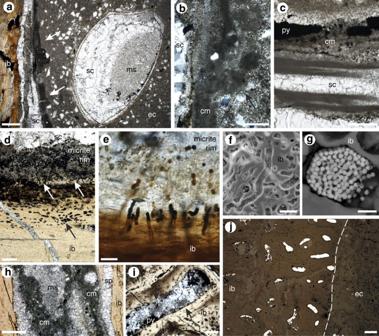Figure 3: Microscale analysis of theOphthalmosaurusbones. (a) Bone covered by a peloidal crust (arrows). The bones are enclosed in a siliciclastic matrix cemented by microsparite. In the right side of the photo, articulated bivalve filled with secondary sparry calcite and microsparite. (b) Detail of the peloidal crust, made by clotted micrite and loosely spaced micritic peloids (arrows). (c) Detail of the peloidal crust. Clotted micrite and pyrite in the upper part; elongated mats representing calcified biofilms in the lower part. (d) Fossil bone extensively bioeroded (white arrows point to microborings), showing a thick micrite rim on the outer side. Bone lacunae are filled with pyrite (black arrow). (e) Close-up of the bioeroded area where microborings are perpendicular to the external bone surface. (f) Empty, elongated microboring. (g) Microboring filled with a pyrite framboid. (h) Cancellous bones filled with clotted micrite, microsparite and sparry calcite. (i) Clotted micrite, pyrite and microbial peloids (arrows) filling the voids of cancellous bones. (j) Pyrite filling cancellous bones decreases in abundance towards the bone centre, and is rare in the surrounding concretion. All transmitted light photomicrographs in plane-polarized light except (j) in reflected light; (f) SEM (scanning electron microscope) image in secondary electron mode, (g) SEM in backscattered electron mode. ib, ichthyosaur bone; sc, sparry calcite; ms, microsparite; ec, enclosing concretion; cm, clotted micrite; py, pyrite. Scale bars, (a) 500 μm; (b,h,j) 200 μm; (c,d,i) 100 μm; (e) 20 μm; (f) 10 μm; (g) 2 μm. Full size image Figure 3: Microscale analysis of the Ophthalmosaurus bones. ( a ) Bone covered by a peloidal crust (arrows). The bones are enclosed in a siliciclastic matrix cemented by microsparite. In the right side of the photo, articulated bivalve filled with secondary sparry calcite and microsparite. ( b ) Detail of the peloidal crust, made by clotted micrite and loosely spaced micritic peloids (arrows). ( c ) Detail of the peloidal crust. Clotted micrite and pyrite in the upper part; elongated mats representing calcified biofilms in the lower part. ( d ) Fossil bone extensively bioeroded (white arrows point to microborings), showing a thick micrite rim on the outer side. Bone lacunae are filled with pyrite (black arrow). ( e ) Close-up of the bioeroded area where microborings are perpendicular to the external bone surface. ( f ) Empty, elongated microboring. ( g ) Microboring filled with a pyrite framboid. ( h ) Cancellous bones filled with clotted micrite, microsparite and sparry calcite. ( i ) Clotted micrite, pyrite and microbial peloids (arrows) filling the voids of cancellous bones. ( j ) Pyrite filling cancellous bones decreases in abundance towards the bone centre, and is rare in the surrounding concretion. All transmitted light photomicrographs in plane-polarized light except ( j ) in reflected light; ( f ) SEM (scanning electron microscope) image in secondary electron mode, ( g ) SEM in backscattered electron mode. ib, ichthyosaur bone; sc, sparry calcite; ms, microsparite; ec, enclosing concretion; cm, clotted micrite; py, pyrite. Scale bars, ( a ) 500 μm; ( b , h , j ) 200 μm; ( c , d , i ) 100 μm; ( e ) 20 μm; ( f ) 10 μm; ( g ) 2 μm. Full size image The most common macroscopic trace fossils on the bone surfaces, found especially on ribs ( n =18), comprise repeating, overlapping sets of five grooves radiating out from a single point, each set with an average diameter of 4 mm ( Fig. 2b,c ; ref. 20 ). These are assigned to the ichnospecies Gnathichnus pentax , which is attributed to the grazing activities of regular echinoids [22] . Extant echinoids graze hard substrates to consume endolithic or surficial organisms such as annelids, sponges, bacteria and algae [23] . In modern whale falls and hydrocarbon seeps, echinoids are frequently observed grazing on bacterial mats [10] , [24] , [25] . Thus, the presence of G. pentax on these Ophthalmosaurus bones is interpreted as the first record of the activities of mat-grazing echinoids in a marine reptile fall community. Microbially mediated products and processes The carbonate concretion enclosing the bones contains grains of quartz, feldspar and biotite mica, and abundant bioclasts (bivalves, ostracods and echinoid spines) in a microsparitic carbonate matrix ( Fig. 3a ). A 200–600-μm-thick dense crust of clotted micrite and loosely spaced micritic peloids covers the outer surfaces of the bones ( Fig. 3a–c ). The peloids have irregular, blurred rims ( Fig. 3b ) and an average diameter of 100 μm. They are interpreted as microbial bioproducts precipitated on the surface of bacterial clumps [26] , or may alternatively represent faecal pellets of mat-grazing polychaetes or gastropods ( cf. ref. 27 ). Elongated, 20-μm-thick, micrite laminae, subparallel to the bone surface ( Fig. 3c ) are interpreted as calcified biofilms [28] . The crust, as a whole, represents a calcified algal or microbial mat that was probably made by variety of microbes that includes filamentous phototrophic and heterotrophic bacteria, and algae, whose activity determine mat calcification and preservation [28] . Its autochthonous formation by in situ calcification is indicated by the purity of the micrite, rarity of intraclasts and its protrusive outer margins [27] . The Ophthalmosaurus bone surface is intensively bioeroded by microborings with an average diameter of 3.7 μm and a maximum measured length of 81.8 μm ( Supplementary Fig. 1 ). They comprise non-bifurcating, straight or slightly curved microtunnels, which are empty or filled by pyrite framboids and preferentially orientated perpendicular to the external bone surface ( Fig. 3d–g ). The mean thickness of the bioeroded zone is 460 μm. Externally, where the density of microborings is the highest, the original bone structure has been replaced by a microcrystalline (micrite) rim containing microtunnel outlines ( Fig. 3d,e ). These are the first such microborings recorded from ichthyosaur bones, although similar examples have been described from modern and fossil whale, sirenian and plesiosaur bones and attributed to cyanobacteria, actinobacteria, algae or fungi [29] , [30] , [31] , [32] , [33] , which are the most common and widespread borers of calcium apatite [34] . Attributing microborings to specific shallow water, endolithic borers is difficult based on morphology alone, because of convergent evolution of boring and reproductive behaviour among unrelated organisms that exploit similar environments [35] . While we cannot exclude the action of actinobacteria, able to degrade bone collagen [33] , we attribute these examples to the activities of cyanobacteria for two key reasons. First, penetration depth is very shallow, as with photosynthetic microborers where penetration of the dark substratum is strongly limited by the depth of light penetration [36] . Second, the presence of a micrite rim on the outer surfaces of the microbored Ophthalmosaurus bones ( Fig. 3d,e ) is consistent with the boring activities of endolithic cyanobacteria, during which Ca 2+ ions are transported along the tricomes to the outer surface of the substrate where they are excreted to form a pure, micritic, poorly crystalline layer [37] . Internally, the cancellous ichthyosaur bones are filled with three carbonate phases: (a) microcrystalline calcite (micrite), (b) patchily distributed microsparite and (c) a sparry, secondary calcite filling the fractures ( Fig. 3h ). The microcrystalline calcite has a clotted fabric ( Fig. 3h ), and locally comprises rounded to sub-rounded peloids, 50–120 μm in diameter ( Fig. 3i ). Clotted textures and peloids are interpreted as being microbial in origin, and are similar to those described from a variety of different geological settings [27] , as well as fossil whale falls [31] , [33] , [38] and upper Cretaceous plesiosaur falls [7] . Thus, we infer that microbial decay of the Ophthalmosaurus bone marrow lipids induced the precipitation of calcium carbonate, which in turn induced the calcification of bacterial aggregates forming the clotted fabric and peloids. Increased availability of reactive organic matter promotes the formation of hydrogen sulphide through anoxic bacterial reduction of seawater sulphate [39] , and a by-product is elevated alkalinity and the precipitation of carbonate minerals. The microsparite cement filling the remaining marrow cavities may then have crystallized around these bacterial aggregates ( cf. ref. 33 ). Pyrite framboids, or iron oxides that retain a framboidal shape ( Supplementary Figs 2 and 3 ), are abundant within the cancellous bones ( Fig. 3i,j ). Their average diameter is 1.91 μm, with most (73.5%) ranging between 0.50 and 3.00 μm ( Supplementary Fig. 1 ). Pyrite framboids are most common towards the outer edge of the bones and decrease in abundance towards the bone centre ( Fig. 3j ). Bone lacunae are also frequently filled with pyrite ( Fig. 3d ). The high concentration of pyrite found in the bone trabeculae is interpreted as being the result of anaerobic microbial decomposition of the bone organic compounds (for example, lipids) and sulphate reduction, which led to the local release of sulphide, as observed in modern and fossil whale falls [38] , [40] , [41] . The rarity of pyrite in the surrounding concretion ( Fig. 3j ) suggests that sulphides formed when the bones were just below the sediment surface (see ref. 39 ), and not during burial diagenesis. Associated invertebrate macrofaunal community In the concretionary blocks, various fossil macroinvertebrates are closely associated with the bones ( Figs 4 and 5 ). Epifaunal suspension feeders dominate the assemblage (61% of the total number of individuals), and the most abundant ( n =55) are shells of the cemented Ostraeidae Deltoideum delta ( Fig. 5a ). Other epifaunal suspension feeders include the cemented serpulid Serpula sulcata ( n =2) and byssate forms, such as the pectinid Camptonectes auritus ( n =11; Fig. 5b ), and the Anomiidae cf. Placunopsis radiata ( n =1). Shallow infaunal suspension feeders (27%) are represented by the common Corbulomima suprajurensis ( n =28; Fig. 5d ), found mostly with articulated valves, and the rare cf. Isocyprina sp. ( n =3; Fig. 5c ); semi-infaunal bivalves are represented by Modiolus bipartitus ( n =3). Also infaunal deposit feeder gastropods of the species Dicroloma trifida ( n =2) were found. Spines of the regular echinoid Rhabdocidaris sp. ( n =8; Fig. 5e ) were found close to the bones, and it is likely that the grazing activities of this taxon produced the trace fossil G. pentax . 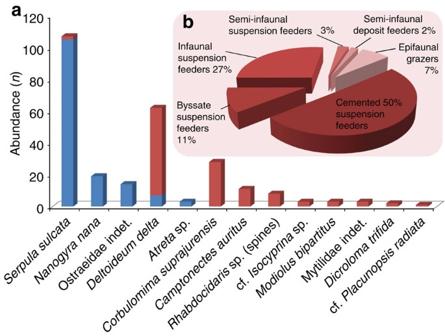Figure 4: Abundance data of macroinvertebrates associated with theOphthalmosaurusbones. (a) Encrusting, suspension-feeding, epibionts on the surface of the bones (in blue); macroinvertebrates close to the bones in the enclosing concretion (in red). (b) Trophic categories of macroinvertebrates in the enclosing concretion; suspension feeders dominate the assemblage. Figure 4: Abundance data of macroinvertebrates associated with the Ophthalmosaurus bones. ( a ) Encrusting, suspension-feeding, epibionts on the surface of the bones (in blue); macroinvertebrates close to the bones in the enclosing concretion (in red). ( b ) Trophic categories of macroinvertebrates in the enclosing concretion; suspension feeders dominate the assemblage. 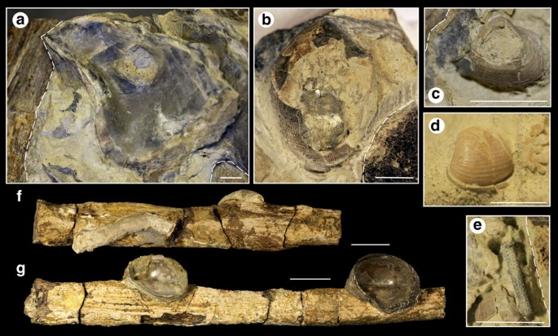Figure 5: Macroinvertebrates associated with theOphthalmosaurusbones. (a)D. delta.(b)C. auritus. (c) cf.Isocyprinasp. (d)C. suprajurensis. (e)Rhabdocidarissp. spine. (f) Rib encrusted byS. sulcata. (g) Rib encrusted byN. nana. Fossil bones outlined by a white, dashed line. Sale bars, (a–c,e–g) 1 cm; (d) 0.3 cm. Full size image Figure 5: Macroinvertebrates associated with the Ophthalmosaurus bones. ( a ) D. delta. ( b ) C. auritus . ( c ) cf. Isocyprina sp. ( d ) C. suprajurensis . ( e ) Rhabdocidaris sp. spine. ( f ) Rib encrusted by S. sulcata . ( g ) Rib encrusted by N. nana . Fossil bones outlined by a white, dashed line. Sale bars, ( a – c , e – g ) 1 cm; ( d ) 0.3 cm. Full size image The overall fossil assemblage is similar to the Nanogyra nana–D. delta association of the overlying lower Kimmeridge Clay [42] , but C. suprajurensis is much more abundant in the ichthyosaur fall assemblage (comprising 24% of the individuals). Similarly, abundant corbulids have been recorded in a Pliocene outer shelf whale fall community [43] . Corbulids are small, infaunal, suspension-feeding r -strategists, thriving in muddy bottoms enriched in organic matter and temporarily depleted in oxygen [44] , [45] . The pectinid C. auritus is also more common around the bones than in the background community. Pectinids are frequently found in modern and fossil shallow-water whale falls [12] , [46] , and are among the most tolerant bivalves to low-oxygen conditions (for example, ref. 47 ). Thus, the relatively high abundances of Corbulomima and Camptonectes may indicate local hypoxia and elevated organic matter flux during microbial decay of the ichthyosaur remains. Encrusting, suspension-feeding epibionts are cemented to some of the bones ( Figs 4 and 5 ). S. sulcata is the most abundant identifiable taxon ( n =105; Figs 4 and 5f ), followed by N. nana ( n =19; Figs 4 and 5g ), D. delta ( n =7) and the plicatulid Atreta sp. ( n =3). They occur on both pristine bones and on bones with echinoid-grazing traces. Ribs and vertebrae were preferentially colonized (20–25% are encrusted) with respect to other bones, such as paddle elements and neural spines (<10%). These encrusting epibionts were probably exploiting flow enhancement, and similar associations have been recorded in fossil ichthyosaur and whale fall assemblages [6] , [12] . The late Oxfordian ichthyosaur fall studied herein supported a wide range of micro- and macro-organisms during the time it was exposed on the seafloor prior to final burial. Comparison with modern whale falls primarily relies on an ecological approach, because evolutionary history has resulted in significant taxonomic differences between modern and Late Jurassic invertebrate marine communities. A critical assumption is that the ichthyosaur bones contained sufficient lipid content to potentially support development of long-lived chemosynthetic communities during a ‘sulphophilic stage’, as in modern and fossil whale falls. Their streamlined morphology and large eyes, especially in the genus Ophthalmosaurus , indicate that ichthyosaurs were able to cruise fast and dive deep [16] . Their cancellous and spongy bones are similar only to those of cetaceans and some large marine turtles that also frequent the deeper portion of the water column [17] . Histological studies of modern marine mammals indicate that reduced bone density is linked to an increase in lipid storage that enables reduced gas retention in the body, resulting in more energy-efficient dives [18] , and it is likely that ichthyosaurs developed the same adaptation. Thus, ichthyosaur carcasses could potentially have supported chemosymbiotic communities similar to those of modern and fossil whale falls. As in whale fall communities, succession was initiated by ‘mobile scavengers’, as evidenced by the tooth marks left on the bones by small fishes. The defleshed, exposed bones were subsequently colonized by a diverse microbial community. Some, such as heterotrophic microbes, would have directly exploited the remaining ichthyosaur organic matter, including lipids from within the bones themselves and the bone collagen, releasing hydrogen sulphide into the local environment. Others colonized the freshly exposed bone surfaces where microbial succession led to the development of a complex and diverse mat community of heterotrophic and photoautotrophic bacteria that spanned the bone–water interface, which in turn attracted invertebrate grazers such as sea urchins and peloid-producing organisms such as polychaetes or gastropods, as in modern whale falls [10] (‘microbial mat and grazer stage’). The abundant encrusting suspension feeders recorded in this study indicate a well-developed ‘reef stage’. This contrasts to the situation in modern [10] and fossil [12] whale falls, where epibiont colonization is patchy. The size of the encrusters indicates that some bones were exposed for at least several years. In modern whale falls, a fully developed ‘reef stage’ has not been recorded due, in part, to the destructive activities of the highly specialized, bone-eating worm Osedax that colonize vertebrate bones from coastal to abyssal depths [48] . Dense Osedax populations are able to consume an entire whale skeleton within a few years [25] , even if in areas of low levels of oxygen their action might be hindered, resulting in skeletons exposed on the seafloor for many decades (for example, ref. 9 ). No trace fossils attributed to Osedax were recorded in this study, which is consistent with phylogenetic analyses that indicate at most a late Cretaceous origin of the Osedax clade [48] and with an early Oligocene age for the oldest known Osedax trace fossil [49] . In the absence of Osedax , bone destruction in Jurassic seas would have been slower than in modern sea, and only burial by sediment would have curtailed development of a ‘reef stage’ in ichthyosaur fall communities. Elucidating the nature of the ecological succession in the sediments surrounding the bones is more difficult owing to low sedimentation rates and the effects of time averaging within the taphonomically active zone. The shallow-water, muddy sediments at the study site probably already supported a benthic macroinvertebrate community prior to the arrival of the dead ichthyosaur. During its decay, environmental conditions close to the carcass may have changed substantially, which would have in turn affected the composition of the local benthic community. The high abundance of corbulids and pectinids probably reflect these changes, indicating elevated organic matter flux and local, transient hypoxia during microbial decay of the ichthyosaur remains. Their presence might thus indicate the development of an ‘enrichment-opportunist stage’ that in modern whale falls is mainly represented by soft-bodied organisms. The absence of any chemosymbiotic macroinvertebrates on or near the bones indicates that anaerobic microbial decay of the bone lipids, testified by the abundant pyrite deposition in the cancellous bones, did not result in a well-developed ‘sulphophilic stage’. While obligate whale-fall chemosynthetic bivalves originated in the Paleogene, others, including the families Lucinidae and Nucinellidae, have an evolutionary history that dates back to the Jurassic and older [50] and therefore potentially could have been associated with the Ophthalmosaurus. Lucinids have been described from offshore, Upper Jurassic seep carbonates from Southern France [51] and the Antarctic [52] , and in the latter example other taxa considered obligate to chemosynthetic habitats have been also found, including hokkaidoconchid gastropods, an extinct family related to the modern whale fall, seep- and vent-dwelling Provannidae [52] . The absence of chemosynthetic taxa associated with the Ophthalmosaurus thus, might be due to the relatively small size of the specimen (estimated at ca. 3 m) and insufficient biomass to sustain a chemosynthetic ecosystem, as in juvenile whale falls [9] . It may also be due to the shelf setting, however, as in shallow-water whale falls the ‘sulphophilic stage’ is rare [10] , [11] , [12] , [13] and the benthic taxa depend principally for their nutrition on carbon fixed by photosynthesis, as in other shallow-water-reducing environments such as hydrothermal vents and cold seeps [53] . The emerging picture is that in the Jurassic, hydrocarbon seeps hosted symbiont-bearing invertebrates [51] , [52] , whereas organic falls, only known from shelf settings so far, did not. Similar to our case study, a shallow-water Ophthalmosaurus from the Callovian Lower Oxford Clay (United Kingdom) supported an encrusting ‘reef stage’ of serpulids and oysters, and was associated with deposit-feeding nuculanoid bivalves and micro-carnivorous scaphopods, but no chemosynthetic taxa [6] . Likewise, Bathonian outer shelf wood fall associations described from Poland were mostly colonized by encrusting oysters and serpulids, with non-obligate gastropods and bivalves and no chemosynthetic fauna [54] . Taphonomic studies of the largest known ichthyosaurs, from the Late Triassic of the western USA, similarly report no associated chemosynthetic taxa [55] . To date, the only examples of chemosynthetic-based communities at organic falls in the Mesozoic are thus restricted to the Upper Cretaceous, with provannid gastropods and vetigastropods associated with plesiosaurs carcasses [7] and chemosymbiotic xylophagian bivalves associated with sunken wood [56] described from outer shelf and slope sediments of Japan. It appears that the interval between the Late Jurassic and Late Cretaceous was critical for the evolution of chemosynthetic organic fall communities. It is probably no coincidence that molecular phylogenies of important chemosynthetic taxa suggest a Cretaceous origin for the crown group [57] . Our study demonstrates that prior to final burial, Late Jurassic shallow-water ichthyosaur falls fulfilled similar ecological roles to shallow-water whale falls. Ecological succession included a ‘mobile scavenger stage’, a possible ‘enrichment-opportunist stage’, a ‘microbial mat and grazer stage’ and a prolonged ‘reef stage’, with the latter stages likely overlapping. Some sulphate reduction occurred within the bones, possibly due to decay of bone lipids, but a lengthy ‘sulphophilic stage’ did not develop and the ichthyosaur fall supported no chemosynthetic taxa. All known pre-Cretaceous shallow-water organic falls appear to have supported non-endemic faunas, with food webs based mainly on photosynthetic, rather than chemosynthetic, carbon. Studied specimen The studied specimen was excavated in 1991 in Dorset, UK, during construction of the A303 Zeals-Bourton bypass [58] . Approximately 55% of the ribs were recovered ( n =70), along with vertebrae ( n =40), vertebral processes ( n =11), paddle elements ( n =38), other limb bones ( n =2) and skull elements ( n =7). It is now curated in the Bristol City Museum and Art Gallery (BRSMG Ce16719). Palaeoecological analysis All of the associated macroinvertebrates and trace fossils that were (a) preserved on the bone surfaces and (b) preserved on the surface of the concretionary blocks, within 10 cm distance from the bones, were counted and identified. All fossils were identified at the finest taxonomic level possible, following [59] , [60] , [61] , and their life habits and diet were assigned according to Wignall [42] . Petrographic microfacies analysis Bone fragments partially enclosed in the carbonate concretion were selected for petrographic microfacies analyses. Ten uncovered, polished petrographic thin sections (30 μm thick) were analysed via an optical light microscope in transmitted and reflected light, using a Nikon eclipse LV100POL microscope equipped with a Nikon DSFil digital camera with NIS-Elements BR imaging software. Selected portions of the thin sections were etched in an aqueous solution of 1% HCl between 10 and 30 s, air dried and C-coated for scanning electron microscope observations and element analysis (scanning electron microscopy-energy-dispersive X-ray spectroscopy). The analyses were carried out with a JEOL JSM-6610 LV scanning electron microscope equipped with a AzTEC EDS for element identification. The operating conditions of the scanning electron microscopes were 5–20 keV accelerating voltage for imaging, and 15–20 keV for elemental analyses. How to cite this article: Danise, S. et al. Ecological succession of a Jurassic shallow-water ichthyosaur fall. Nat. Commun. 5:4789 doi: 10.1038/ncomms5789 (2014).